A strategic approach to recharging lithium-sulphur batteries for long cycle life The success of rechargeable lithium-ion batteries has brought indisputable convenience to human society for the past two decades. However, unlike commercialized intercalation cathodes, high-energy-density sulphur cathodes are still in the stage of research because of the unsatisfactory capacity retention and long-term cyclability. The capacity degradation over extended cycles originates from the soluble polysulphides gradually diffusing out of the cathode region. Here we report an applicable way to recharge lithium-sulphur cells by a simple charge operation control that offers tremendous improvement with various lithium-sulphur battery systems. Adjusting the charging condition leads to long cycle life (over 500 cycles) with excellent capacity retention (>99%) by inhibiting electrochemical reactions along with severe polysulphide dissolution. This charging strategy and understanding of the reactions in different discharge steps will advance progress in the development of lithium-sulphur batteries. To satisfy the demand for efficient energy storage employed in electric vehicles, smart energy grids and renewable energies, development of next-generation battery systems is an inevitable task for researchers. Lithium-ion (Li-ion) batteries have been widely applied in consumer electronics successfully for over two decades, and are being developed for other purposes in electric vehicles, aerospace devices and military applications. Research in high-energy-density battery systems including lithium-sulphur (Li-S) and Li-air batteries is critical for developing next-generation thinner, lighter and lower-cost battery systems [1] . Following the cell design of commercialized Li-ion batteries, Li-S cells with solid-state sulphur cathodes are expected to receive fewer challenges than Li-air batteries with gaseous cathodes [1] , [2] . As the insulating issue of sulphur/lithium sulphide (Li 2 S) can be solved by the incorporation of conductive carbon materials, the main obstacle that remains in the Li-S battery is the dissolution of polysulphide intermediates produced during electrochemical reactions [2] , [3] , [4] . Much work has been reported to address this problem by trapping dissolved active materials in the cathode matrix; however, capacity fade is still observed even after these diverse approaches. 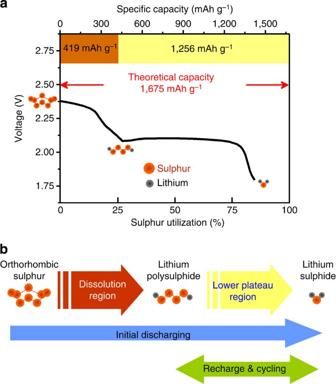Figure 1: Recharge strategy for elongating the cycle life of Li-S batteries. (a) Typical discharge profile of the Li-S battery showing an upper plateau and a lower plateau. (b) The strategic approach to recharge Li-S batteries. A full initial discharge followed by recharging and cycling within the lower plateau region. The lower plateau possesses a theoretical capacity of 1,256 mAh g−1. As seen in Table 1 , many advanced Li-S battery systems have been designed and have shown remarkable progress [5] , [6] , [7] , [8] , [9] , [10] , [11] , [12] , [13] . For example, high capacities of >1,000 mAh g −1 (based on sulphur weight) during initial cycles and longer cycle life (>100 cycles) have been demonstrated. Nevertheless, in most cases, the discharge capacity tends to gradually decay with increasing cycle number and time. To gear the Li-S battery research towards practical applications, other approaches should be adopted to integrate with the currently developed electrodes/systems. Table 1 Summary of the performance of advanced Li–S battery systems. Full size table Constraining the charge capacity or voltage window of Li-ion batteries has been widely applied for stabilizing the cathode reactions for years. For instance, LiCoO 2 cathodes cannot be charged to more than 50% of their theoretical capacity (140 mAh g −1 ); otherwise, oxygen loss from the lattice will occur leading to chemical and structural instabilities [14] . In industry, safe operating charge/discharge voltages are defined according to the stable electrochemical reaction region in the battery system to avoid overcharge/overdischarge, which might cause electrode and electrolyte decomposition. The Li-S battery is usually operated between 2.8 and 1.5 V. If lithium nitrate (LiNO 3 ) is added in the electrolyte for improving the Coulombic efficiency, the terminal discharge potential should be raised to over 1.7 V to prevent the irreversible reduction of LiNO 3 (refs 4 , 15 ). Herein we develop a simple recharge technique that can significantly enhance the cycle life of Li-S cells under long-term and repeated cycling conditions. By recharging the cell within the lower plateau (Li 2 S↔Li 2 S 4 (predominant); theoretical capacity: 1,256 mAh g −1 , see Fig. 1a ), the battery performance can be improved considerably with a fade-free cyclability. The upper plateau involves oxidation–reduction reactions between soluble long-chain polysulphides and sulphur (Li 2 S 4 ↔S (predominant); theoretical capacity: 419 mAh g −1 ), where the well-known shuttle effect occurs significantly, especially during charging [4] , [16] , [17] . Although the kinetics of these redox reactions are very fast [18] , obvious capacity fading is still found on prolonged cycles or during slow charging/discharging, even with state-of-the-art electrode designs. The reason is that when the charge/discharge processes cover the highly unstable dissolution region (the upper plateau), a small fraction of the active material migrates out of the electrode during every cycle and it may not be utilized again. Moreover, the highly reactive polysulphide anions could react with the electrolyte solvent, resulting in a depletion of the electrolyte [4] ; therefore, gradual capacity degradation is seen. Our approach exhibited in Fig. 1b is to confine the predominant electrochemical reactions to the lower potential plateau region between insoluble Li 2 S and soluble Li 2 S 4 . It should be noted that the ‘lower plateau region’ here represents the production/consumption of the solid-phase Li 2 S, not all-solid-state reaction since Li 2 S 4 can dissolve in the electrolyte. In fact, Li 2 S 4 has smaller solubility in ether-based electrolytes than other long-chain polysulphide intermediates [19] , which can effectively reduce the severe dissolution behaviour of active material. The solid-state active material (Li 2 S) is present, at least a certain amount, at all stages during cycling, facilitating not only the precipitation of Li 2 S (serving as nuclei) but also the adsorption of soluble lithium polysulphides (serving as an adsorbent). Therefore, the outward diffusion of soluble long-chain polysulphides from the cathode is negligible, leading to highly stable capacity output for hundreds of cycles. Figure 1: Recharge strategy for elongating the cycle life of Li-S batteries. ( a ) Typical discharge profile of the Li-S battery showing an upper plateau and a lower plateau. ( b ) The strategic approach to recharge Li-S batteries. A full initial discharge followed by recharging and cycling within the lower plateau region. The lower plateau possesses a theoretical capacity of 1,256 mAh g − 1 . Full size image Electrochemical performance with modified recharge setting The cycle performance comparison between the cells with the regular recharge setting (charging to 2.8 V) and the modified recharge setting (charging until reaching 600 or 1,000 mAh g −1 ) is shown in Fig. 2a . Stable electrochemical reactions can be accomplished as long as the charge capacity is controlled within the lower plateau region ( Supplementary Fig. S1 ). These cells were assembled with a microporous carbon interlayer configuration, which can significantly enhance the active material utilization and cyclability at high rates [20] . However, we found that when the Li-S batteries with interlayers were cycled under a lower C rate, capacity fading behaviour can be observed during long-term cycling. The first discharge capacity of the cell under the regular recharge condition is as high as 1,483 mAh g −1 at C/5 rate (335 mA g −1 ), but it declines to less than 1,000 mAh g −1 before the 100th cycle. In contrast, the cells under the modified recharge condition outputs stably the discharge capacity with almost exactly the same value up to 300 cycles. The capacity degradation rates of the cells charged until reaching 600 and 1,000 mAh g −1 are, respectively, only 0.0011 and 0.0027% per cycle, which are an order of magnitude lower than the best record reported by Seh et al. [5] . This evidence further confirms that the upper plateau reactions are the main causes of the performance deterioration in the Li-S cell system. Accordingly, a simple recharge modification can play a critical role in the stabilization of electrochemical reactions for the sulphur cathode in the Li-S battery. 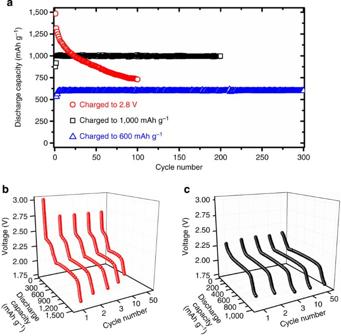Figure 2: Cycle performance of the Li-S batteries with the modified recharge setting. (a) Cycle performance of the Li-S cells with the regular recharge setting (charging to 2.8 V) and the modified recharge setting (charging to 1,000 or 600 mAh g−1) at C/5 rate. (b) Discharge curves of the Li-S cell with the regular recharge setting at various cycles. (c) Discharge curves of the Li-S cell with the modified recharge setting (charging to 1,000 mAh g−1) at various cycles. Figure 2: Cycle performance of the Li-S batteries with the modified recharge setting. ( a ) Cycle performance of the Li-S cells with the regular recharge setting (charging to 2.8 V) and the modified recharge setting (charging to 1,000 or 600 mAh g −1 ) at C/5 rate. ( b ) Discharge curves of the Li-S cell with the regular recharge setting at various cycles. ( c ) Discharge curves of the Li-S cell with the modified recharge setting (charging to 1,000 mAh g −1 ) at various cycles. Full size image Figure 2b and Supplementary Fig. S2a display the discharge profiles of the cell with the regular recharge setting. As seen, the upper plateau keeps shrinking with increasing cycle number, implying that the utilizable active material gradually decreases. In fact, the length of the lower plateau is also shortened as cycling proceeds owing to the loss of soluble polysulphides. To ensure the Li-ion transport between the electrolyte and the cathode region, the electrode should possess adequate channels for lithium ions to pass through; otherwise, the electrochemical reactions will terminate owing to insufficient ion supply followed by lack of electron exchange. Therefore, the long-chain polysulphides formed in the dissolution region might still migrate out of the cathode slowly and cannot be recaptured by the porous structure in the following cycles. While charging the cell within the lower plateau region, the concern of active material loss from serious polysulphide dissolution is eliminated. In Fig. 2c and Supplementary Fig. S2b , the discharge profiles of the cell recharged to 1,000 mAh g –1 majorly possess the 2-V plateau. Although a part of the sloping region can be seen after cycling, it occupies only a small portion of about 10–15% of the whole discharge profile. This affirms that the redox reactions can be preferentially selected by controlling the charging parameters. All of the lower plateaus at various cycles perform well with the discharge capacity close to 1,000 mAh g −1 , representing an extraordinarily stable electrochemical reaction under this recharge operation. Even in the primitive Li-S battery, the cell with the capacity-controlled recharge setting still outperforms the one with the traditional recharge setting, which decays drastically during the initial five cycles ( Supplementary Fig. S3 ). The capacity value of the initial lower discharge plateau determines the maximum charge capacity that can be realized with stable cyclability, so a well-utilizable sulphur cathode is preferred to couple with this recharge strategy. It should be noted that although we performed the cycling by limiting the cutoff charge capacity, the voltage of the cell cycled by limiting the cutoff charge capacity to 600 mAh g −1 increased only from 2.34 to 2.38 after 500 cycles, indicating negligible increase in polarization during cycling. Polysulphide species verified by ex situ XPS measurements To further understand the impact of different polysulphide formations on battery performance, ex situ X-ray photoelectron spectroscopic (XPS) analysis of the interlayer samples retrieved from cycled cells was carried out without exposing the samples to air by employing an air-sensitive sample transfer chamber. Earlier reports have constructed a complete redox reaction mechanism of Li-S batteries via impedance analysis [21] , in situ X-ray diffraction [22] , [23] , ex situ scanning electron microscopy [21] , [22] , [24] , ultraviolet–visible absorption spectroscopy [25] and liquid chromatography [25] , [26] . Various XPS analyses have been carried out to investigate the Li electrode surface [27] , [28] but in-depth XPS measurements have not been conducted for detecting specific polysulphides separately so far. To avoid the side reactions between polysulphides and electrolyte during cell resting, a higher C rate of C/2 was used as the discharge rate for the XPS samples to assure the polysulphide intermediates are majorly produced from electrochemical reactions. Pristine sulphur and Li 2 S powder, which have the binding energy of, respectively, 163.7 and 159.8 eV were measured beforehand as the references ( Supplementary Fig. S4 ). 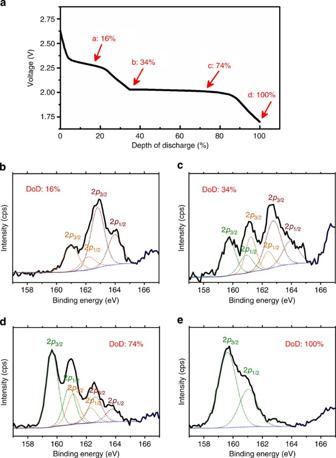Figure 3:Ex situXPS measurements of cycled interlayers. (a) Discharge curve of the Li-S cell cycled at C/2 rate with the depth of discharge (DoD) indicated. XPS plots of the active material at (b) 16% DoD, (c) 34% DoD, (d) 74% DoD and (e) 100% DoD. (2p3/2-brown(Li2S6): 162.8 eV; 2p3/2-yellow(Li2S4): 161.2 eV; and 2p3/2-green(Li2S): 159.8 eV). Figure 3 displays a series of XPS results at different depths of discharge (DoD, Fig. 3a ). The peaks with the binding energy over 168 eV contributed by lithium trifluoromethanesulphonate (LiCF 3 SO 3 ) can be found in all samples ( Supplementary Fig. S5 ) [29] . Near the end of the upper plateau (DoD=16%, Fig. 3b ), two lithium polysulphide peaks were detected. At the beginning of the lower plateau (DoD=34%, Fig. 3c ), not only the previous two polysulphide peaks are observed but also a small pure Li 2 S peak is recognized. This finding is quite distinct from the mainstream electrochemical redox mechanisms that claim Li 2 S 2 is formed before the end product Li 2 S. However, the XPS data show that Li 2 S, with the same binding energy as the pristine Li 2 S powder, is generated immediately after the start of the lower plateau, and this will be discussed in the following paragraph. At the middle of the lower plateau (DoD=74%, Fig. 3d ), three XPS peaks are still detected but with different intensities, representing the consumption of the higher-valent active polysulphides and the formation of Li 2 S. At the end of the lower plateau (DoD=100%, Fig. 3e ), unsurprisingly, only Li 2 S is observed as the major product. From the recent work of Diao et al. [26] , Li 2 S 6 and Li 2 S 4 are found as the most stable form of Li 2 S n compounds in the Li-S battery, so the first polysulphide with high binding energy in Fig. 3b could be Li 2 S 6 and the second one with low binding energy in Fig. 3b must be Li 2 S 4 according to the combined capacity of the upper plateau and the sloping region (~419 mAh g –1 ) [18] , [26] . It should be noted that the number in the chemical formula of polysulphides here only represents their average oxidation state. Figure 3: Ex situ XPS measurements of cycled interlayers. ( a ) Discharge curve of the Li-S cell cycled at C/2 rate with the depth of discharge (DoD) indicated. XPS plots of the active material at ( b ) 16% DoD, ( c ) 34% DoD, ( d ) 74% DoD and ( e ) 100% DoD. (2 p 3/2-brown (Li 2 S 6 ): 162.8 eV; 2 p 3/2-yellow (Li 2 S 4 ): 161.2 eV; and 2 p 3/2-green (Li 2 S): 159.8 eV). Full size image In fact, early Li-S battery studies stated that Li 2 S 2 is stable in solid phase, yet it has not been fully confirmed in the sulphur cathode [24] , [30] . Another early report claimed that Li 2 S 2 is the main product of the lower plateau by the output capacity from the battery, but not by materials characterization [31] . Until now, there is no convincing proof from X-ray diffraction showing the existence of Li 2 S 2 but only Li 2 S after discharging [21] , [22] , so the species of Li 2 S 2 might not dominate the battery reactions in this case. Barchasz et al. [25] applied ultraviolet–visible spectra to the determination of various polysulphides in Li-S cells, and the authors did observe the presence of S 8 2− , S 6 2− , S 3 ·− , S 5 2− , S 4 2− , S 3 2− , S 2 2− and S 2− . Nevertheless, several polysulphide species originate from the disproportionation reactions but not redox reactions. In contrast, the samples were measured in the form of catholyte, which might lead to different reaction mechanisms compared with ours. From former ex situ scanning electron microscopic analysis, solid-phase active material forms right after the beginning of the lower plateau reactions in accordance with the Li 2 S detection in our report [21] , [22] . In addition, the migration of active material from its original location in carbon-based cathodes due to the polysulphide dissolution was observed [21] , [22] , [24] . Li 2 S 6 formed at the end of the upper plateau is found as a highly soluble lithium polysulphide from the observation of the electrolyte colour [29] , [32] , which is possibly the most unwanted soluble species in solid-state Li-S cells. By uniting the scientific reports above, we propose here a probable concise reaction mechanism for Li-S batteries in Fig. 4 . At a moderate or high cycling rate, the Li-S battery shows a three-step profile, the upper plateau, the sloping region and the lower plateau, and each part represents the formation of predominate active materials, which are, respectively, Li 2 S 6 , Li 2 S 4 and Li 2 S. Moreover, the polysulphide intermediates dissolved in the electrolyte are always a mixture and they cannot be in the form of a single compound [26] . The discharge mechanism of Li-S cells with the dioxolane/dimethoxyethane-based electrolyte is then clarified, although this may need to be modified for different electrolytes [33] , active material concentrations [25] , electrode designs [13] and charge/discharge rates. 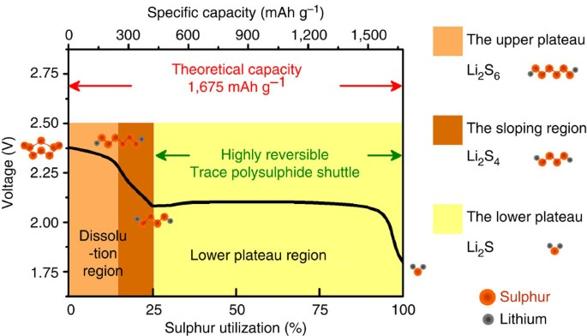Figure 4: The discharge reaction mechanism of a Li-S battery. The discharge profile can be divided into three regions: the upper plateau, the sloping region and the lower plateau. The former two are located in the dissolution region, and the latter is located in the lower plateau region that provides highly reversible capacity and has only a negligible amount of polysulphide shuttle behaviour. Figure 4: The discharge reaction mechanism of a Li-S battery. The discharge profile can be divided into three regions: the upper plateau, the sloping region and the lower plateau. The former two are located in the dissolution region, and the latter is located in the lower plateau region that provides highly reversible capacity and has only a negligible amount of polysulphide shuttle behaviour. Full size image Cells with LiNO3-free electrolyte with the recharge strategy LiNO 3 has been widely applied in Li-S cells to enhance Coulombic efficiency since it was found to passivate the Li anode and thus prevent the polysulphide shuttle attack [15] , [27] , [28] . However, LiNO 3 can be irreversibly reduced on the cathode surface, resulting in the instability of electrochemical reactions [15] . There are also safety concerns with LiNO 3 because of its strong oxidative property [4] . Furthermore, using this additive in the electrolyte may give researchers a misleading impression that battery systems work perfectly once they obtain high Coulombic efficiency. Here we also tested the cell with the interlayer but filled with a LiNO 3 -free electrolyte to illustrate this point. 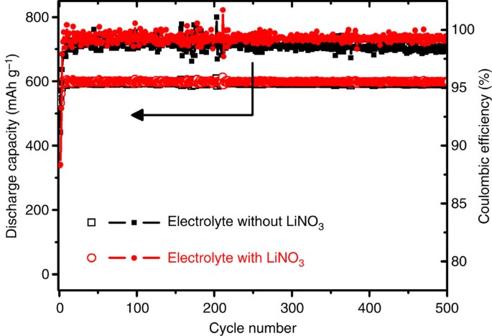Figure 5: Impact of LiNO3additive on battery performance with the recharge strategy. The LiNO3-free electrolyte is also suitable for Li-S cells to obtain high Coulombic efficiency by utilizing the modified recharge setting. The C rate applied here was C/5. Figure 5 compares the influence of the LiNO 3 additive in the electrolyte on the Coulombic efficiency of the cell with the modified recharge setting. Even without the assistance of LiNO 3 , the Li-S battery still has an efficiency of as high as 98.1% after 500 cycles, implying that the lower plateau reaction is highly reversible with minimal energy loss during charging. In other words, the long-standing polysulphide shuttle issue can be solved because of the suppression of the long-chain polysulphide production by employing our recharge strategy. Figure 5: Impact of LiNO 3 additive on battery performance with the recharge strategy. The LiNO 3 -free electrolyte is also suitable for Li-S cells to obtain high Coulombic efficiency by utilizing the modified recharge setting. The C rate applied here was C/5. Full size image Li/dissolved polysulphide cells with modified recharge setting To determine whether this recharge setting is applicable to various Li-S battery systems, another promising Li/dissolved polysulphide (Li 2 S 6 ) battery with a binder-free carbon nanofibre (CNF) electrode, which is similar to our recent work with carbon nanotube electrodes, was cycled by only charging within the lower plateau region [29] . The microstructure of the low-cost CNF mat is shown in Supplementary Fig. S6 , which has an interwoven network that can trap the active material. It can be seen in Supplementary Fig. S7 that the initial discharge curve has only the sloping region and the lower plateau. Note that there is no upper plateau in this cell because the starting active material is Li 2 S 6 instead of pristine sulphur. Therefore, Li 2 S 6 should be generated right before the sloping region in a regular Li-S cell, and this behaviour is in agreement with the assumed discharge mechanism we mentioned before. 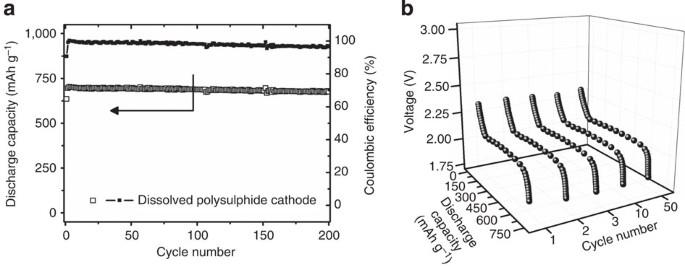Figure 6: Li/dissolved polysulphide cells with the modified recharge setting. (a) Cyclability, Coulombic efficiency and (b) discharge curves of the Li/dissolved polysulphide cell using commercial CNF electrode with the modified recharge setting (charging to 700 mAh g−1) at C/5 rate. Figure 6a shows the extended cycling results of the Li/dissolved polysulphide cell. The discharge profiles of the battery after the 1st, 2nd, 3rd, 10th and 50th cycles are exhibited in Fig. 6b and Supplementary Fig. S8 . These output capacities, which are contributed from the single plateau at near 2 V, are exactly similar. The superior cycle stability proves that the developed recharge setting can be broadly applied to different battery designs for elongating the cycle life of Li-S cells. Figure 6: Li/dissolved polysulphide cells with the modified recharge setting. ( a ) Cyclability, Coulombic efficiency and ( b ) discharge curves of the Li/dissolved polysulphide cell using commercial CNF electrode with the modified recharge setting (charging to 700 mAh g −1 ) at C/5 rate. Full size image In summary, the main cause of the deteriorating performance of Li-S batteries can be ascribed to the irreversible upper plateau reactions. Utilizing only the lower plateau during cycling significantly extends the cell cycle life, which can be realized via a simple modified recharge setting. By charging the Li-S battery within the lower plateau capacity, high capacity and long cyclability with an ultra-low capacity degradation rate of 0.0011% per cycle (~0.53% for 500 cycles here) can be readily obtained, which is the best capacity retention recorded in the literature at this time. The lower plateau near 2 V involves the reaction directly forming insoluble Li 2 S confirmed by air-sensitive XPS analysis. In addition, various lithium polysulphide products are detected in the upper plateau and sloping regions, and these soluble species could migrate/react irreversibly in the absence of Li 2 S, leading to strong shuttle effect and capacity fade. Moreover, the co-salt of LiNO 3 in the electrolyte will be unnecessary to improve the Coulombic efficiency if this recharge strategy is applied. This modified recharge approach is not only feasible with the Li-S cells with an interlayer configuration but also is viable with the dissolved polysulphide systems. We believe this recharge modification could be widely applied with various electrode designs and cell systems, thereby advancing the practical use of Li-S batteries for high-performance energy storage. Preparation of Li-S cells with microporous interlayers Cathode slurry was prepared by mixing 70 wt% pristine sulphur, 20 wt% conductive carbon black (Super P) and 10 wt% polyvinylidene fluoride (Kureha) polymer binder with N -methylpyrrolidinone (Sigma-Aldrich) as a mixing medium overnight. The sulphur-contained slurry was coated onto an aluminium current collector sheet by the tape-casting method and then dried for 24 h at 50 °C in air, followed by roll pressing and cutting into circular disks. The sulphur loading in the cathode disk is around 1.5–1.7 mg cm −2 . The microporous interlayers were fabricated by mixing commercial high-surface-area carbon black with abundant micropores (Black Pearls 2000, CABOT) and polytetrafluoroethylene polymer binder at a 60:40 weight ratio. These materials were mixed in a mortar with a small amount of isopropyl alcohol as a mixing medium, followed by roll pressing and cutting into circular disks. Both cathode disks and microporous interlayers with about the same mass of the cathode were dried in a vacuum oven for an hour at 50 °C before cell assembly. The electrolyte was prepared by dissolving the appropriate amount of LiCF 3 SO 3 , 98% (Acros Organics) and LiNO 3 , 99+% (Acros Organics) in a 1,2-dimethoxyethane (99+%, Acros Organics) and 1,3-dioxolane (99.5%, Acros Organics; 1:1 v/v) mixture to render a 1.85 M LiCF 3 SO 3 and 0.1 M LiNO 3 solution. LiNO 3 -free electrolyte was prepared by using 1.85 M LiCF 3 SO 3 as the only lithium source in the electrolyte. The CR2032 coin cells were assembled in the sequence of sulphur cathodes, prepared electrolyte, microporous interlayers, polypropylene separators (Celgard 2400) and lithium metal anodes (Aldrich) in an Argon-filled glove box. Finally, the cell was crimped and took out of the glove box for electrochemical evaluation. Preparation of Li/dissolved polysulphide cells The process of fabricating the self-weaving CNF mat is similar to our previous approach [34] . Commercial CNFs with curly structure (150 mg, Sigma-Aldrich) were dispersed in 750 ml of deionized water by high-power ultrasonication for 15 min with the addition of 20 ml of isopropyl alcohol to wet the CNFs. The products were collected by vacuum filtration and washed with deionized water, ethanol and acetone for several times. The free-standing CNF paper thus formed was a flexible film after drying for 24 h at 100 °C in air, which can be easily peeled off the filter membrane. The blank electrolyte used in the Li/dissolved polysulphide system was with 1 M LiCF 3 SO 3 salt instead of 1.85 M employed with the interlayer configuration. To prepare the dissolved polysulphide catholyte, sublimed sulphur powder (99.5%, Acros Organics) and an appropriate amount of lithium sulphide (Li 2 S, 99.9%, Acros Organics) were added to the appropriate amount of blank electrolyte to render 1.5 M sulphur in the form of Li 2 S 6 in the solution. The mixture solution was heated at 45 °C in an Ar-filled glove box for 18 h to produce a dark yellow solution with moderate viscosity. Li/dissolved polysulphide in CR2032 coin cells were assembled in an Ar-filled glove box. First, 40 μl of polysulphide catholyte was added into the CNF paper electrode, corresponding to 1.9 mg (1.7 mg cm −2 ) of sulphur. Then a Celgard separator was placed on the top of the CNF electrode. A volume of 20 μl of blank electrolyte was added onto the separator, followed by the lithium metal anode. Finally, the cell was crimped and took out of the glove box for electrochemical evaluation. Battery test The discharge/charge profiles and cyclability data were obtained with a programmable battery cycler (Arbin Instruments). The C rates specified in this study are based on the mass and theoretical capacity of sulphur (1,675 mA g −1 ). The batteries after cell assembly were rested for an hour before the cycling test. In a regular charge setting, the cell was discharged/charged in the voltage window of 2.8—1.7 V. In a modified charge setting, all of the cells were fully discharged during the initial cycle, followed by being recharged until reaching a certain value of charge capacity based on the experimental designs. The cells for XPS measurements were fully cycled for several times, and discharged until reaching specific DoD and then stopped by the cycler program. Air-sensitive XPS analysis The samples were examined by XPS with a Kratos Axis Ultra spectrometer (Kratos Analytical) utilizing a monochromated Al Kα X-ray source ( hν =1486.5 eV) and a 45° take-off angle. The pressure in the analysis chamber was typically 2 × 10 −9 torr during data acquisition. The microporous interlayer proved to be an efficient polysulphide trap in the Li-S cell, so it was used to analyse the polysulphide intermediates at different DoD. The unwashed interlayers were extracted from independent coin cells within an argon-filled glove box with the H 2 O and O 2 concentrations of <0.1 p.p.m. and transferred to the spectrometer right away via a custom interface (built at the Surface Analysis Laboratory of the Texas Materials Institute at the University of Texas at Austin) to avoid hydrolysis or oxidation of Li 2 S and lithium polysulphides. The residue electrolyte was evaporated during the vacuum processing. Details of the design of the interface will be published elsewhere. All spectra were fitted with Gaussian–Lorentzian (30% Gaussian) functions and a Shirley-type background by the deconvolution software (CasaXPS, Casa Software). Three constraints on the component peaks were applied: the position (1.18 eV between S 2 p 3/2 and S 2 p 1/2 ), the peak area ratio (S 2 p 3/2 :S 2 p 1/2 =2: 1) and equal full width at half maximum. All reported binding energy values are calibrated to the graphitic C 1 s peak with a value of 284.5 eV and the peak of sulphate signal from the LiCF 3 SO 3 residue with a value of 169.7 eV. How to cite this article: Su, Y.-S. et al. A strategic approach to recharge lithium-sulphur batteries for long cycle life. Nat. Commun. 4:2985 doi: 10.1038/ncomms3985 (2013).